Notch1–Dll4 signalling and mechanical force regulate leader cell formation during collective cell migration At the onset of collective cell migration, a subset of cells within an initially homogenous population acquires a distinct ‘leader’ phenotype with characteristic morphology and motility. However, the factors driving the leader cell formation as well as the mechanisms regulating leader cell density during the migration process remain to be determined. Here we use single-cell gene expression analysis and computational modelling to show that the leader cell identity is dynamically regulated by Dll4 signalling through both Notch1 and cellular stress in a migrating epithelium. Time-lapse microscopy reveals that Dll4 is induced in leader cells after the creation of the cell-free region and leader cells are regulated via Notch1–Dll4 lateral inhibition. Furthermore, mechanical stress inhibits Dll4 expression and leader cell formation in the monolayer. Collectively, our findings suggest that a reduction of mechanical force near the boundary promotes Notch1–Dll4 signalling to dynamically regulate the density of leader cells during collective cell migration. Collective cell migration is a fundamental multicellular activity that plays essential roles in numerous physiological and pathological processes, such as embryogenesis, tissue regeneration and cancer metastasis [1] , [2] , [3] , [4] . Proper coordination of cells, for instance, is required to repair damaged tissues in which the cells crawl collectively atop exposed extracellular matrix following injury. The collective migration mechanisms responsible for embryogenesis and tissue repair are also utilized in the invasion and metastasis of malignant tumours [3] , [5] . For instance, collective invasion of squamous cell carcinomas in the form of clusters or stands is often observed in histopathological analyses [6] , [7] . A known mechanism of collective migration is ‘purse string’ closure, where a multicellular actin bundle formed among cells at the boundary of a small wound draws the wound together [8] , [9] . Another mechanism of collective cell migration is the formation of migration tips [3] ( Fig. 1a ). Migration tips with leader–follower organization are observed in the healing of larger wounds and cancer invasion. In particular, specialized leader cells appear at the leading edge and exert mechanical force on follower cells [10] , [11] . In an organotypic co-culture invasion model, fibroblasts serve as leaders to drive the collective migration of carcinoma cells [12] . Remarkably, integrins α3 and α5 along with myosin light-chain activity in fibroblasts are required for force-mediated matrix remodelling; however, these factors are not required in the trailing carcinomas, suggesting biomechanical coupling and a leader–follower organization in the invasion process. 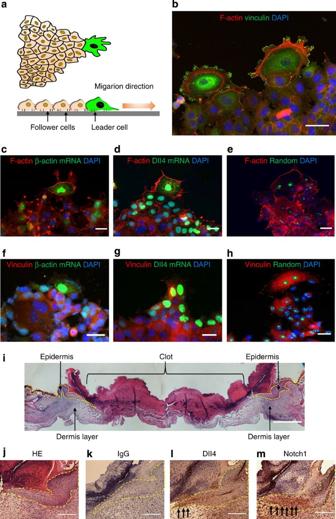Figure 1: Characteristics of leader cells in collective cell migration. (a) Schematic representation of a migration tip with leader–follower organization during collective cell migration. Leader cells (green) at the front of the leading edge typically display enlarged cell size, ruffling lamellipodium, large focal adhesions and aligned cytoskeletal architecture. (b) Representative immunofluorescence image of F-actin (red) and vinculin (green) in leader cells formed at the leading edge. (c–e) Actin stress fibres in cells transfected with dsLNA probes targeting (c) β-actin mRNA, (d) Dll4 mRNA and (e) a random sequence. Cells were first transfected with the dsLNA probes (green) and fixed for immunostaining (red). (f–h) Focal adhesion in cells transfected with dsLNA probes targeting β-actin mRNA (f), Dll4 mRNA (g) and a random sequence (h). Samples were counterstained with DAPI (blue). Images are representative of three independent experiments. Scale bars, 50 μm. (i–j) HE staining of epithelial cells in skin punch wounds. (k–m) IHC staining of IgG control (k), Dll4 (l) and Notch1 (m). Yellow dotted lines indicate the epithelium and black arrows indicate the wound boundaries. Scale bars, 200 μm. Figure 1: Characteristics of leader cells in collective cell migration. ( a ) Schematic representation of a migration tip with leader–follower organization during collective cell migration. Leader cells (green) at the front of the leading edge typically display enlarged cell size, ruffling lamellipodium, large focal adhesions and aligned cytoskeletal architecture. ( b ) Representative immunofluorescence image of F-actin (red) and vinculin (green) in leader cells formed at the leading edge. ( c – e ) Actin stress fibres in cells transfected with dsLNA probes targeting ( c ) β-actin mRNA, ( d ) Dll4 mRNA and ( e ) a random sequence. Cells were first transfected with the dsLNA probes (green) and fixed for immunostaining (red). ( f – h ) Focal adhesion in cells transfected with dsLNA probes targeting β-actin mRNA ( f ), Dll4 mRNA ( g ) and a random sequence ( h ). Samples were counterstained with DAPI (blue). Images are representative of three independent experiments. Scale bars, 50 μm. ( i – j ) HE staining of epithelial cells in skin punch wounds. ( k – m ) IHC staining of IgG control ( k ), Dll4 ( l ) and Notch1 ( m ). Yellow dotted lines indicate the epithelium and black arrows indicate the wound boundaries. Scale bars, 200 μm. Full size image Leader cells are usually identified by their distinct morphologies [10] , [13] , [14] . These specialized leader cells display enlarged cell size, ruffling lamellipodium, large focal adhesions and aligned cytoskeletal architecture. Recently, basal epithelial genes, including cytokeratin 14 (K14) and p63, were observed in leader cells in an organoid breast cancer invasion assay [15] . Several other genes, such as β-actin, Erk1/2 and RhoA, are also upregulated near the boundary [16] , [17] , [18] . In addition, mechanical force and Rho signalling have been suggested to influence leader cell formation. External compressive stress, disruption of the tensile actomyosin cable with two-photon photoablation, geometric cues with contact printing and modulation of Rho signalling were shown to influence leader cells [10] , [11] , [18] , [19] , [20] . Furthermore, exchanging leaders in the invading front was observed in breast cancer cells in collagen gel [21] . Nevertheless, it is not known how leader cells are initiated among the initially homogeneous population, nor is it known how leader cell density is dynamically regulated during collective migration. In this study, we investigate the initiation, regulation and function of leader cells during collective cell migration using single-cell gene expression analysis in conjunction with computational modelling. We apply time-lapse microscopy to track the formation and evolution of leader cells by monitoring the expression of a Notch ligand, delta-like ligand 4 (Dll4). Dll4 was originally identified in the arterial endothelium [22] . Notch1–Dll4 lateral inhibition dynamically regulates the ratio between tip cells and stalk cells in response to angiogenic factors by restricting excessive tip cell formation during angiogenic sprouting [23] , [24] . Nevertheless, the involvement of Dll4 in leader cell formation during epithelialization has not been studied. We therefore examine the level of Dll4 along with other leader cell characteristics, and monitor the initiation and distribution of leader cells during collective migration. A wound-healing assay and single-cell photothermal ablation are applied to study the evolution of leader cells and their functions [25] , [26] . Using a combined experimental and computational approach, the interplays of Notch1–Dll4 signalling and intercellular force in the emergence of leader cells are investigated. Dll4 is a molecular signature of leader cells To investigate leader cells, we applied a double-stranded locked nucleic acid (dsLNA) assay for detecting gene expression at the single-cell level [17] , [27] , [28] and compared the acquired gene expression with other leader cell characteristics. Leader cells are typically characterized by their phenotypes, including enlarged morphology and active lamellipodium on the migration tip. Leader cells also develop well-defined vinculin-based focal adhesions and reorganize cortical actin into peripheral actin cables and stress fibres ( Fig. 1b ). We performed the dsLNA assay and immunostaining simultaneously to correlate leader cell characteristics with the expression of β-actin and Dll4 mRNAs ( Fig. 1c–h and Supplementary Fig. 1a ). Enlarged leader cells with enhanced actin stress fibres near the leading edge exhibited high levels of β-actin mRNA ( n =15; Fig. 1c ). In contrast, follower cells were smaller and displayed a low level of β-actin mRNA. The expression of β-actin mRNA also correlated with the formation of focal adhesions and lamellipodia in leader cells ( n =10). Large, distinct focal adhesions were observed at the migrating front of leader cells expressing high levels of β-actin mRNA ( Fig. 1f ). Non-leader cells at the boundary, however, had only a few focal adhesions and low levels of β-actin mRNA. We also studied the expression of Dll4, which is expressed in endothelial cells during angiogenesis [22] , [23] . Remarkably, the level of Dll4 mRNA was significantly upregulated in the tips of the migrating epithelium, but not in other cells at the boundary or in the inner region of the monolayer ( n =20; Fig. 1d,g and Supplementary Fig. 1a ). Similar to β-actin mRNA, Dll4 mRNA also correlated with the formation of stress fibres and focal adhesions. Time-lapse microscopy further indicated that cells with high Dll4 mRNA levels displayed distinct morphologies with enlarged cell size and ruffling lamellipodium at migration tips ( Supplementary Movie 1 ). Examining the random probe, which had a low intensity, confirmed the specificity of the assay and the insignificant effect of the probe on cell migration ( Fig. 1e,h and Supplementary Fig. 1b,c ). Furthermore, haematoxylin–eosin (HE) staining and immunohistochemistry (IHC) were performed in mouse skin punch wounds to investigate the expression of Dll4 near the wound boundary. HE staining indicated the morphology of epithelium cells near the wound ( Fig. 1i,j ) and IHC staining showed the expression of Dll4 and Notch1 in epithelial cells ( Fig. 1k–m ). Both Dll4 and Notch1 were upregulated near the wound boundary. We further characterized the distribution of leader cells near the boundary ( Supplementary Fig. 2 ). The intensity levels of β-actin and Dll4 at the leading edge (that is, the first row) did not follow a Gaussian distribution and were better described by using bimodal distributions. The leader cell subpopulation with distinctively high levels of β-actin and Dll4 mRNAs represented ~25% of cells at the leading edge. The intensity levels of HO-1 probes and random probes, on the contrary, displayed smooth Gaussian-like distributions at the leading edge. The distinct subpopulations observed, therefore, were unlikely due to the enlarged size or additional uptake of probes by the leader cells. We further analysed the spatial distribution of gene expression at subsequent rows from the boundary. The average intensity and the number of cells with distinctively high β-actin and Dll4 mRNA signal decreased significantly in the second row of cells. The varying intensities of the cells resembled Gaussian distributions in the third and fourth rows of cells for both probes, indicating that leader cells are spatially regulated. In agreement with previous studies [17] , HO-1 mRNA were upregulated near the boundary. However, the intensity of HO-1 probe showed smooth, Gaussian-like distribution at all positions, similar to the leading edge. The intensity of random probe also maintained a low level regardless of location relative to the leading edge. Taken together, these results indicate that Dll4 and β-actin are molecular signatures of leader cells. Dynamic regulation of leader cells via Notch1–Dll4 signalling The dsLNA probe for Dll4 mRNA allowed us to track the initiation and evolution of leader cells. The Dll4 expression of leader cells was monitored near the boundary using time-lapse microscopy ( Supplementary Movie 1 ). The formation of leader cells was highly dynamic. Leader cells with upregulated Dll4 mRNA and motile phenotypes were detected ~4 h after wounding. Dll4 upregulation was primarily observed near the boundary ( Fig. 2a ). The majority of leader cells were initiated from the first row (>80%), although they occasionally originated from the second row ( n =30 and Supplementary Fig. 3a ). Tracking the Dll4 expression revealed the diverse behaviour of cells. While some cells near the leading edge increased Dll4 expression after wounding, other cells decreased or maintained their level of Dll4 ( Fig. 2b ). The latter behaved as followers during migration. Interestingly, a portion (~10%) of cells transiently increased the Dll4 expression, with the expression decreasing eventually to basal level ( Fig. 2c and Supplementary Fig 3b ). 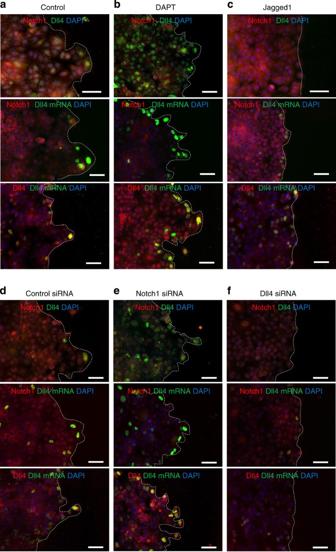Figure 3: Notch1–Dll4 signalling regulates leader cell formation in collective cell migration. (a–c) Double immunofluorescence staining of Notch1 and Dll4 in model wounds (top). For Dll4 mRNA detection, cells were first transfected with the dsLNA probes before fixation for Notch1 and Dll4 immunostaining (middle and bottom). (a) Notch1 nuclear translocation and Dll4 expression in model wounds. (b,c) Effects of DAPT (b) and Jagged-1 (c) on Notch1 and Dll4 proteins and Dll4 mRNA. (d–f) Effects siRNA knockdown on Notch1 and Dll4 and Dll4 mRNA. Control siRNA (d), Notch1 siRNA (e) and Dll4 siRNA (f) were transfected to the cells 48 h before wounding. Samples were counterstained with DAPI (blue). Images are representative of three independent experiments. Scale bars, 100 μm. 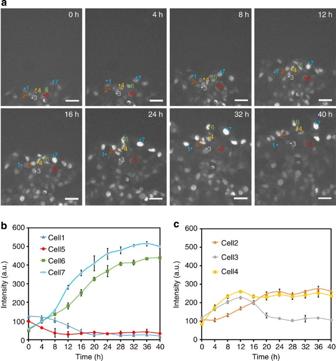These results indicate that the leader cell formation is triggered and regulated dynamically after the creation of the cell-free region. Figure 2: Dynamics of Dll4 expression and leader cell formation during collective migration. (a) Time-lapse fluorescence images characterizing Dll4 mRNA expression. Cells were transfected with dsLNA probes targeting Dll4 mRNA. The model wound was created by scratching the monolayer with a sterilized 1,000 μl pipette tip. Scale bars, 50 μm. Representative cells were labelled with numbers (1–7). (b,c) Tracing of Dll4 mRNA expression in representative cells inaillustrating the dynamic behaviours and competitive characteristics of leader cells in collective migration (n=3). Pixel intensity data are expressed as the mean±s.e.m. Figure 2: Dynamics of Dll4 expression and leader cell formation during collective migration. ( a ) Time-lapse fluorescence images characterizing Dll4 mRNA expression. Cells were transfected with dsLNA probes targeting Dll4 mRNA. The model wound was created by scratching the monolayer with a sterilized 1,000 μl pipette tip. Scale bars, 50 μm. Representative cells were labelled with numbers (1–7). ( b , c ) Tracing of Dll4 mRNA expression in representative cells in a illustrating the dynamic behaviours and competitive characteristics of leader cells in collective migration ( n =3). Pixel intensity data are expressed as the mean±s.e.m. Full size image We studied the roles of Notch signalling in the regulation of leader cells, since Dll4 is a ligand of Notch receptors. We examined the levels of Notch1 and Dll4 protein, as well as their correlation with Notch1 and Dll4 mRNA. Notch1 nuclear translocation was observed in a region ~300 μm from the leading edge and displayed a random distribution in the inner monolayer ( Fig. 3a and Supplementary Figs 4a and 5a ). Leader cells expressed both Dll4 mRNA and Dll4 protein, further supporting the notion that Dll4 is a molecular signature of leader cells. In contrast, cells in the monolayer expressed a low level of Dll4 protein. These observations were in agreement with IHC staining. To further study the roles of Notch signalling, cells were treated with a γ-secretase inhibitor, DAPT ( Fig. 3b and Supplementary Figs 4b and 5b ). With DAPT treatment, which inhibits Notch receptor cleavage and signalling, Notch1 mRNA and protein expressions were reduced in cells, suggesting autoregulation of Notch1. Furthermore, the number of leader cells with elevated Dll4 mRNA and protein increased at the boundary. In contrast, treatment with Jagged-1, a Notch ligand, increased the levels of Notch1 mRNA and protein. This observation further supports the autoregulation of Notch1. The number of leader cells was reduced as indicated by the Dll4 expression, the cell morphology and the density of migration tips ( Fig. 3c and Supplementary Figs 4c and 5c ). Figure 3: Notch1–Dll4 signalling regulates leader cell formation in collective cell migration. ( a – c ) Double immunofluorescence staining of Notch1 and Dll4 in model wounds (top). For Dll4 mRNA detection, cells were first transfected with the dsLNA probes before fixation for Notch1 and Dll4 immunostaining (middle and bottom). ( a ) Notch1 nuclear translocation and Dll4 expression in model wounds. ( b , c ) Effects of DAPT ( b ) and Jagged-1 ( c ) on Notch1 and Dll4 proteins and Dll4 mRNA. ( d – f ) Effects siRNA knockdown on Notch1 and Dll4 and Dll4 mRNA. Control siRNA ( d ), Notch1 siRNA ( e ) and Dll4 siRNA ( f ) were transfected to the cells 48 h before wounding. Samples were counterstained with DAPI (blue). Images are representative of three independent experiments. Scale bars, 100 μm. Full size image We also investigated the involvement of Notch1–Dll4 signalling in the formation of leader cells using short interfering RNA (siRNA). The efficiencies of Notch1 siRNA and Dll4 siRNA were evaluated by immunoblotting ( Supplementary Fig. 6 ) [29] , [30] . Notch1 siRNA significantly reduced the Notch1 protein compared with control siRNA ( Fig. 3d,e and Supplementary Fig. 4d,e ). Notch1 siRNA also increased Dll4 at both mRNA and protein levels and promoted the formation of migration tips. Furthermore, Dll4 siRNA diminished the expression of Dll4 mRNA and protein ( Fig. 3f and Supplementary Fig. 4f ). Dll4 siRNA also suppressed the formation of leader cells and migration tips. Overall, these results support the notion that Notch1 signalling inhibits Dll4 at the leading edge and regulates the density of leader cells. Notch and mechanical force regulate leader cell formation Traction force microscopy has suggested a tug-of-war model with a gradient of cellular stress near the boundary [31] , [32] , [33] . We studied the effects of mechanical force on Dll4 expression and the regulation of leader cells. We confirmed the gradient of cellular stress in our experimental conditions by traction force microscopy ( Supplementary Fig. 7 ). We then studied the effects of cell traction force on leader cell formation. ROCK inhibitor Y-27632 and myosin inhibitor blebbistatin, which reduce the cell traction force [34] , significantly increased the number of leader cells expressing Dll4 at the leading edge ( Fig. 4a and Supplementary Fig. 8 ). The leader cells displayed invasive phenotypes and a large number of migratory tips are formed at the boundary. In contrast, cells treated with calyculin-A or nocodazole, which increase the cell traction force [35] , [36] , reduced the number of Dll4 expressing cells and the number of migration tips significantly, supporting the idea that cellular stress inhibits the formation of leader cells ( Fig. 4a ) [18] . 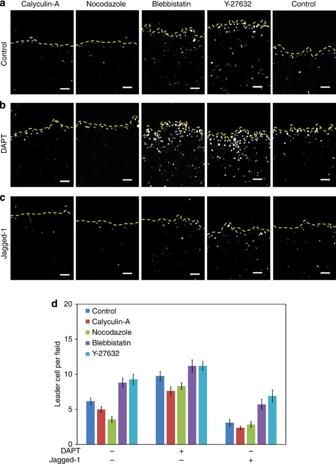Figure 4: Mechanical force and Notch signalling regulates the formation of leader cells. (a) Effects of traction force-modulating reagents on Dll4 mRNA expression near the leading edge. Cells were transfected with dsLNA to detect the distribution of Dll4. (b,c) Effects of co-treatment of DAPT (b) or Jagged-1 (c) and cellular force-modulating reagents on Dll4 expression and leader cell formation. Yellow dotted lines indicate the leading edges. Images are representative from three independent experiments. Scale bars, 100 μm. (d) Density of Dll4-expressing leader cells at the leading edges. Data are expressed as mean±s.e.m. (n=3). Figure 4: Mechanical force and Notch signalling regulates the formation of leader cells. ( a ) Effects of traction force-modulating reagents on Dll4 mRNA expression near the leading edge. Cells were transfected with dsLNA to detect the distribution of Dll4. ( b , c ) Effects of co-treatment of DAPT ( b ) or Jagged-1 ( c ) and cellular force-modulating reagents on Dll4 expression and leader cell formation. Yellow dotted lines indicate the leading edges. Images are representative from three independent experiments. Scale bars, 100 μm. ( d ) Density of Dll4-expressing leader cells at the leading edges. Data are expressed as mean±s.e.m. ( n =3). Full size image To study the interplay between cellular stress and Notch signalling, DAPT and Jagged-1 were co-treated with the force-modulating reagents. DAPT treatment increased the number of leader cells in all conditions near the boundary ( Fig. 4b,d ). Strikingly, a large number of cells in the inner region of the monolayer expressed Dll4 when DAPT was co-treated with Y-27632 or blebbistatin. Leader cells were not observed in the inner region of the monolayer when cells were treated with DAPT, Y27632, or blebbistatin alone. In contrast, the number of Dll4-expressing cells in the inner region significantly decreased with DAPT co-treated with force inducers, calyculin-A or nocodazole. Jagged-1, on the other hand, reduced the formation of leader cells in all force-modulating reagents ( Fig. 4c,d ). Collectively, the spatial distribution of Dll4 expression suggests a coupling between mechanical force and Notch1–Dll4 signalling. These results propose that while traction force can play an essential role in initiating leader cell formation, the Notch signalling pathway is responsible for modulating the leader cell density in collective migration. Thus, the reduction of cellular stress, due to the gradient of traction force near the boundary, promotes Dll4 expression and leader cell formation. Computational modelling of leader cell formation We further investigated the relationship between cellular stress and Notch1–Dll4 lateral inhibition in leader cell formation using a computational model ( Supplementary Note 1 ). The in silico model incorporated Notch1–Dll4 lateral inhibition and force-dependent Notch activity to predict the Dll4 expression near the boundary. For Notch-Dll4 lateral inhibition, initial random fluctuations of the Notch1 and Dll4 levels in cells at the leading edge could lead to stable patterns of gene expression. In particular, a Dll4-expressing leader cell induces the Notch1 level in neighbouring cells, creating spatial patterns of Dll4 expressing leader cells with approximately equal spacing ( Supplementary Movie 2 ). Furthermore, Notch1 and Dll4 expression was modelled as a function of the cellular stress near the boundary, which was supported by traction force microscopy and force-modulating experiments. The incorporation of the force dependence in Notch1–Dll4 activity captured the Dll4 distribution ( Fig. 5a ) and the diverse dynamic behaviour of Dll4 expression ( Fig. 5b and Supplementary Movie 3 ). The numerical model also predicted the spatial distribution of Notch1 near the boundary, as observed in immunostaining ( Supplementary Note 1 ). 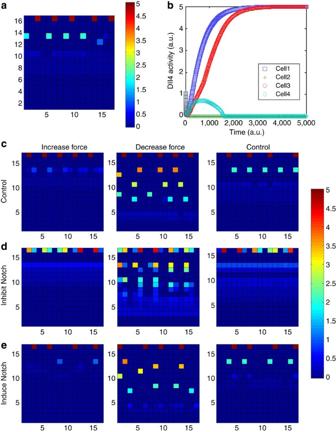Figure 5: Computational modelling of leader cell formation regulated by mechanical force and Notch1–Dll4 lateral inhibition. (a) Representative distribution of Dll4 expressing tip cells from the computational model. (b) Tracking of Dll4 levels in representative cells at the leading edge. Time is in arbitrary units in the computational model. (c–e) Effects of modulating the force distribution and Notch1–Dll4 interaction on leader cell formation. The top boundaries represent the leading edges. The color bars show the level of Dll4 in arbitrary units. Figure 5: Computational modelling of leader cell formation regulated by mechanical force and Notch1–Dll4 lateral inhibition. ( a ) Representative distribution of Dll4 expressing tip cells from the computational model. ( b ) Tracking of Dll4 levels in representative cells at the leading edge. Time is in arbitrary units in the computational model. ( c – e ) Effects of modulating the force distribution and Notch1–Dll4 interaction on leader cell formation. The top boundaries represent the leading edges. The color bars show the level of Dll4 in arbitrary units. Full size image We applied the computational model to study the emergence of leader cells by mechanical force and Notch1–Dll4 lateral inhibition ( Fig. 5c–e ). When the Notch1–Dll4 interaction was reduced, a larger number of Dll4 expressing cells were observed near the boundary and the transient competition of Dll4 was significantly increased ( Fig. 5d ). These results were in good agreement with the DAPT treatment experiment, which inhibited Notch receptor cleavage and signalling, and promoted leader cell formation ( Fig. 4b ). Inducing Notch signalling in the model ( Fig. 5e ), on the other hand, inhibited Dll4 expression and reduced the number of leader cells, similar to the induction of Notch by Jagged-1 ( Fig. 4c ). Furthermore, adjusting the cell traction force in individual cells modulated the distribution of stress and Dll4 in the migrating epithelium. In particular, reducing the cell traction force enhanced the formation of Dll4-expressing cells while increasing the cell traction force reduced the Dll4 level in the inner monolayer ( Fig. 5c–e ). With simultaneous traction force reduction and Notch inhibition, the Dll4 level increased in both the leading edge and the inner region. In contrast, increasing the cell traction force generally reduced the Dll4 expression and inhibited the formation of Dll4-expressing cells in the inner monolayer. These results support the notion that a reduction in mechanical force promotes v signalling to induce leader cell formation during collective cell migration. Photothermal ablation of leader cells We perturbed leader cells to further study their regulations and functions. Single-cell photothermal ablation was performed to disrupt leader cells at the boundary ( Fig. 6a and Supplementary Movie 4 ). Following photothermal ablation, new leader cells with elevated Dll4 mRNA and motile phenotypes were detected after a few hours. The level of Dll4 in the newly formed leader cells continuously increased over 12 h ( Fig. 6b ). To shed light on the function of leader cells, the migration speed of the leading edge was analysed after the disruption of the leader cells ( Fig. 6c ). Remarkably, the speed of the leading edge was reduced dramatically after cell ablation. Nevertheless, the speed gradually increased and reached the control level after 10–12 h. Notably, the time required to regain the initial speed correlated with the timescale of Dll4 expression. In addition, the existence of ablated leader cells could reduce the speed of the leading edge. We therefore performed control experiments to selectively ablate non-leader (random) cells at the boundary ( Fig. 6c ). The migration speed of cells with random cell disruption was significantly higher than those with leader cell disruption in the first 6 h. After the formation of new leader cells, the migrating speeds were similar between random and leader cell disruption. To further study the relationship between leader cell density and the migration speed, we applied DAPT and Jagged-1 to modulate the number of leader cells at the leading edge ( Fig. 7a,b ). We measured the migration speed of cells treated with DAPT or Jagged-1 ( Fig. 7c,d ). Results showed that the migration speed correlated with the density of the leader cells. In particular, DAPT treatment increased the leader cell density and the migration speed. The leader cell density and the migration speed both decreased in Jagged-1 treated cells. 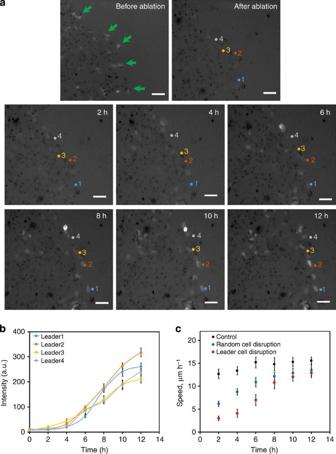Figure 6: Photothermal ablation of leader cells. (a) Photothermal ablation to disrupt leader cells at the leading edge. Leader cells (green arrows) were first identified using dsLNA targeting Dll4 mRNA and ablated using a 1,064-nm fibre laser coupled with GNRs internalized in the cells. Formation of new leader cells was monitored for 12 h after leader cells being disrupted. Results are from three independent experiments. Scale bar, 50 μm. (b) Expression of the Dll4 mRNA in selective cells numbered ina. Pixel intensity data are expressed as the mean±s.e.m. (c) Effects of leader cell ablation and the migration speed of the leading edge. Data are expressed as mean±s.e.m. (n=3). Figure 6: Photothermal ablation of leader cells. ( a ) Photothermal ablation to disrupt leader cells at the leading edge. Leader cells (green arrows) were first identified using dsLNA targeting Dll4 mRNA and ablated using a 1,064-nm fibre laser coupled with GNRs internalized in the cells. Formation of new leader cells was monitored for 12 h after leader cells being disrupted. Results are from three independent experiments. Scale bar, 50 μm. ( b ) Expression of the Dll4 mRNA in selective cells numbered in a . Pixel intensity data are expressed as the mean±s.e.m. ( c ) Effects of leader cell ablation and the migration speed of the leading edge. Data are expressed as mean±s.e.m. ( n =3). 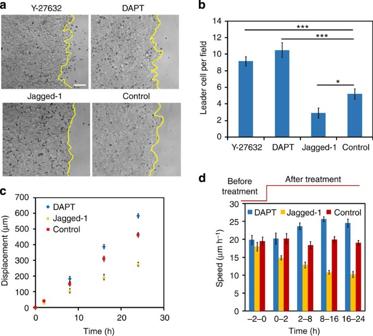Figure 7: Migration speed correlates with leader cell density. (a,b) Bright-field images illustrating the leading edges with Y-27632, DAPT, Jagged-1 and control. Yellow lines indicate the leading edges. Data are expressed as mean±s.e.m. (n=3, *P<0.05, ***P<0.001; unpaired Student’st-test). (c,d) Displacement and collective migration speed of cells at different leader cell densities under the treatment of DAPT and Jagged-1. Data are expressed as mean±s.e.m. (n=3). Scale bar, 100 μm. Full size image Figure 7: Migration speed correlates with leader cell density. ( a , b ) Bright-field images illustrating the leading edges with Y-27632, DAPT, Jagged-1 and control. Yellow lines indicate the leading edges. Data are expressed as mean±s.e.m. ( n =3, * P <0.05, *** P <0.001; unpaired Student’s t -test). ( c , d ) Displacement and collective migration speed of cells at different leader cell densities under the treatment of DAPT and Jagged-1. Data are expressed as mean±s.e.m. ( n =3). Scale bar, 100 μm. Full size image In this study, the essential roles of Dll4 in the formation and regulation of leader cells are identified. Dll4 levels correlate with the phenotypic and morphological markers of leader cells in living cells and mouse skin punch wounds. The ability to monitor Dll4 mRNA in living cells enables us to follow the initiation and regulation of leader cells. Our results suggest that leader cell formation is regulated by Notch1–Dll4 lateral inhibition, as supported by pharmacological treatment, siRNA knockdown, computational modelling and photothermal ablation ( Figs 3 , 4 , 5 , 6 ). This finding provides a molecular basis for the stochastic emergence of leader cells, a process whose regulatory mechanism remained unclear [10] . Computational modelling of Notch1–Dll4 lateral inhibition vindicates the transient dynamics observed in the live-cell-tracking experiments and depicts the spatial distribution of leader cells. Notch1–Dll4 signalling provides an autoregulatory mechanism to maintain the density of leader cells during collective migration. If the density of Dll4-expressing leader cells is high, the Notch1 level in neighbouring cells will be enhanced, in turn inhibiting Dll4 expression. If the leader cell density is low or a leader cell loses its function, as observed in the photothermal ablation experiment, new leader cells will emerge to restore the migration process. In addition, other Notch ligands and receptors may also regulate the formation of leader cells. Further investigation is required to clarify the involvement of other members of the Notch family in the regulation of leader cells. Our results also demonstrate that mechanical stress inhibits Dll4 expression and leader cell formation. The cell-free region, due to wounding, modulates the stress distribution near the boundary as shown by traction force microscopy ( Supplementary Fig. 7 ). Remarkably, a combination of force-reducing agents and Notch inhibitors dramatically increases the number of Dll4-expressing cells, even in the inner region of the monolayer. Reduction of Notch signalling itself, however, does not induce Dll4-expressing cells in the inner region of the monolayer, suggesting the reduction of mechanical force is required to initiate the formation of leader cells. In contrast, enhancing the cellular stress reduces the formation of Dll4-expressing cells. The importance of mechanical force in leader cell formation is consistent with previous studies using external compressive stress [11] , actomyosin disruption [18] , geometric confinement [19] and biochemical modulation of Rho signalling [10] . Our single-cell gene expression analysis directly evaluates the distribution of leader cells. The regulatory role of mechanical force also explains purse string and migration tip mechanisms in wound healing. For a small wound, the assembly of multicellular actin bundles generates mechanical stress to close the wound and inhibit the formation of leader cells. The formation of migration tips, on the other hand, may be advantageous in healing a large area, in which the purse string is not effective for wound closure. In this scenario, the low cellular stress near the boundary promotes the formation of leader cells, which lead migration tips. Our results suggest that reduction in cellular stress promotes Notch1–Dll4 signalling and leader cell initiation at the leading edge. In fact, Notch signalling is shown to be force dependent and mechanical force is required to pull on Notch and expose the ADAM cleavage site for proteolysis and downstream signalling [37] , [38] , [39] . The combination of mechanical force and Notch1–Dll4 lateral inhibition may represent a robust strategy to regulate the collective migration process. During epithelization, the Notch1–Dll4 signalling is induced until the wound is healed and the mechanical stress is restored. This process represents a feedback mechanism for the cells to regulate wound healing. The stress distribution maintains leader–follower organization, which prevents the formation of leader cells behind the migration tip [20] . Furthermore, Notch signalling enables the dynamic regulation of the leader cell density and may explain leader cell exchange in three-dimensional collective migration models [12] , [21] , [40] . The exchange of leader cells is arguably a cooperative strategy enabling cells to maximize their interaction with the local chemical gradient [40] and minimize the thermodynamic cost of migration [21] . Cell culture and reagents dsLNA probes and synthetic targets for calibration were synthesized by Integrated DNA Technologies (San Diego, CA). The probe sequences are available in Supplementary Table 1 . All siRNA were purchased from Qiagen (Valencia, CA). The siRNA sequences are available in Supplementary Table 2 . Nocodazole, blebbistatin and calyculin A were purchased from Sigma (St Louis, MO) and Y27632 was obtained from Calbiochem (San Diego, CA). DAPT and Jagged-1 peptide were purchased from Sigma (Saint Lious, MO) and AnaSpec (San Jose, CA) respectively. All pharmacological agents were dissolved in dimethyl sulfoxide (Sigma). Other chemicals and reagents were purchased from Sigma (Saint Louis, MO), unless otherwise specified. Human mammary epithelial cells (MCF-7) were obtained from ATCC (Manassas, VA). Cells were maintained in Dulbecco’s Modified Eagle’s Medium (DMEM; Invitrogen, Carlsbad, CA) supplemented with 10% fetal bovine serum, 2 mM HEPES buffer and 0.1% gentamycin. Cells were plated either in 24-well tissue culture plates or on glass coverslips placed in six-well plates, and they were incubated at 37 °C with 95% humidity and 5% CO 2 . For wound-healing experiments, cells were seeded at an initial concentration of 10 5 cells ml −1 for 2 days to form a confluent monolayer before wounding. To study the effects of Notch signalling, cell monolayers were treated with 20 μM DAPT or 20 μM Jagged-1 for 12 h before scratching. To evaluate the effects of mechanical force on leader cell formation, cells were incubated with 5 nM calyculin A or 10 μM nocodazole to increase cell traction force; 40 μM blebbistatin or 20 μM Y27632 were alternatively utilized to reduce cell traction force. For siRNA experiments, cells were transfected with siRNA from Qiagen (Valencia, CA, USA) using HiPerFect transfection reagent (Qiagen) following the manufacturer’s instructions. A concentration of 20 pM siRNA was applied 48 h before performing the scratch assay. Animals and treatments Adult male SKH-I mice were fed on laboratory food and tap water ad libitum in a regular 12-h dark/light cycle. The University of Arizona Institutional Animal Care and Use Committee approved all animal work and protocols. Before the wound surgery, the mice were anaesthetized with 1–5% isoflurane. The mice back and neck were cleaned with alcohol swabs and betadine. The mice received subcutaneous pre-surgical analgesia (buprenorphine 0.05 mg kg −1 ) and two 6-mm diameter wounds were made on the back of the neck and the dorsal midline, respectively, by using a sterile 6 mm skin biopsy puncher (Health link, Jacksonville, FL). After the surgery, 3M Tegaderm pads were used to cover the biopsy site. Seven days later, the mice were anaesthetized through intraperitoneal injection of 240 mg kg −1 avertin. The wound area skin tissues (8 mm diameter) were collected and the skin tissues were cut into two halves in the middle for later use. Mouse skin tissue immunohistochemical analysis The mice skin tissues were embedded in paraffin and cut into 4-μm sections for HE and IHC staining. The deparaffinized sections were boiled in sodium citrate buffer (10 mM, PH 6.0) for antigen retrieval of IHC, and the primary antibodies (Dll4 and Notch 1) were used in a dilution of 1:200 for 4 °C overnight. Finally, the envision system HRP-DAB kit (DAKO North America. CA) was used according to the product instruction. Single-cell gene expression analysis in living cells The dsLNA probes were used to monitor the dynamic expression of target mRNAs near the boundary. The design, characterization and assay protocol of the dsLNA probes were described previously [17] , [27] , [28] . A donor probe, which consists of a nucleic acid sequence complementary to the target mRNA, is labelled with a fluorophore (6-FAM) at the 5′ end. A complementary sequence is also designed with a quencher (Iowa Black RQ) placed on the 3′ end. Without a target mRNA, the fluorophore and quencher probes remain in close proximity, diminishing the fluorescence signal. With the presence of a target mRNA, the quencher probe is displaced by the target thermodynamically, allowing the donor probe to fluoresce. In the present study, dsLNA probes consist of alternating LNA/DNA monomers, which improve the intracellular stability and the specificity of the probes [41] . The dsLNA probes were designed based on target mRNA sequences, including β-actin, HO-1, Notch1 and Dll4 ( Supplementary Table 1 ). A random probe, lacking a complementary mRNA, was designed as the negative control. The mRNA sequences were obtained from NCBI GenBank and the dsLNA probe sequences were designed using Mfold and NCBI Basic Local Alignment Search Tool (BLAST). The dsLNA probes were prepared by mixing donor and quencher probe sequences at a 1:2 ratio immediately before transfection. On reaching 90% confluency in 24-well plates, cells were transfected with 0.8 μg dsLNA probe using Lipofectamine 2000 in opti-MEM from Invitrogen (Grand Island, NY) to determine the target gene expression. Gene expression was evaluated by measuring the fluorescence intensity of cells transfected with dsLNA probes. Cell migration assays and time-lapse microscopy To perform the cell migration assay, cell monolayers with or without drug treatment were incubated in 24-well tissue culture plates in serum-free media for 45 min. In the experiment, a 1-mm wide model wound was created by scratching the cell monolayer with a sterilized 1,000 μl pipette tip. In the leader cell formation experiment, cells were refreshed with DMEM containing serum. Time-lapse microscopy with bright-field and fluorescence imaging was performed using a microscope stage-top incubator from Okolab (NA, Italy). For migration assays involving drug treatments, cells were maintained with the same concentration of drugs throughout the experiment, and the migration of the epithelia was monitored after performing the scratch assay. Single-cell photothermal ablation To disrupt the leader cells formed at the monolayer’s leading edge, single-cell photothermal ablation was performed using a 1,064 nm fiber laser coupled with gold nanorods (GNRs) taken up by the cells. The photothermal ablation experiment has been previously optimized for both single-cell ablation and minimizing injury to the neighbouring cells [26] . This was confirmed by monitoring the cell viability, gene expression and cell apoptosis of individual cells [26] . Before the experiment, cells were plated on glass bottom 24-well plates after incubation with 2 × 10 11 GNR ml −1 for 12 h. The scratch assay was performed on the cell monolayer and leader cell formation was monitored with the dsLNA probe specific for Dll4 mRNA. Leader cells were identified and irradiated with a 150-mW laser using a × 40 objective, which focused the laser spot to 15 μm (0.85 mW μm −2 power density). The laser module was attached to the microscope (Nikon, TE2000-U) through an epi-fluorescence port. The plasmonic GNRs absorbed the power of the near-infrared laser and induced localized heating to ablate the cells. Leader cells were ablated in a few seconds. A short irradiation time localized the photothermal effect to the target cells [26] , [42] . Immunofluorescence staining For immunostaining, cells cultured on glass coverslips were fixed with 4% paraformaldehyde in 1 × PBS for 10 min. The cells were then washed three times with PBS for 5 min and permeabilized with 0.1% Triton-X-100 for 8 min. The cells were blocked with either 5% goat serum or 1% bovine serum albumin for 30 min. Rhodamine Phalloidin (Invitrogen Molecular Probes, Eugene, 1:400 dilution) was incubated with cells for 25 min for visualizing the actin cytoskeleton. Primary antibodies against vinculin (Sigma, St Louis, MO, 1:400 dilution), Notch1 and Dll4 (Santa Cruz Biotechnology, Santa Cruz, CA, 1:50 dilution) were incubated at room temperature for 1 h. The binding of primary antibodies was visualized via Alexa Fluor 488- or Alexa Fluor 555-conjugated secondary IgG antibodies with 1 h incubation at room temperature. Nuclei were then stained with DAPI (4',6-diamidino-2-phenylindole) antifade reagent from Invitrogen (Carlsbad, CA). Western blot analysis For immunoblotting, cells were treated with 20 nM of control siRNA, Notch1 siRNA and Dll4 siRNA for 48 h. The protein samples were collected using the RIPA lysis buffer (50 mM Tris-Cl (pH 7.4), 150 mM NaCl, 1 mM EDTA, 1% NP-40, 0.25% Na-deoxycholate, 1 mM PMSF, 10 μg ml −1 aprotinin, 10 μg ml −1 leupeptin, 1 mM Na 3 VO 4 and 1 mM NaF) [43] . The samples were quantified using the BCA protein assay kit (Santa Cruz Biotechnology, CA). Proteins (20 μg per well) were subjected to SDS–polyacrylamide gel electrophoresis (10%, Bio-Rad) and transferred to a PVDF membrane (Santa Cruz Biotechnology, CA). Immunoprobing was performed using a rabbit monoclonal GAPDH antibody (1:1,000), a rabbit monoclonal Notch1 antibody (1:800) and a rabbit polyclonal Dll4 antibody (1:400), followed by binding with horseradish peroxidase-conjugated anti-rabbit antibody (1:1,000). Autoradiography films and western blotting luminol reagent (Santa Cruz Biotechnology, CA) were used for the detection. Traction force microscopy Glass-bottomed Petri dishes (MatTek) were activated with 0.1 M NaOH overnight and silanized with 3-aminopropyl-trimethoxysilane (Sigma) for 10 min. The dishes were then thoroughly washed with deionized water and allowed to dry. For image registration, 300 μl of yellow fluorescent carboxylate-modified particles (2 μm diameter, 1:2,000 diluted, Invitrogen) was added to each activated glass surface and air dried overnight. After treatment with 0.5% glutaraldehyde (Sigma) in PBS for 30 min and several washes with deionized water, the glass substrate was ready for gel attachment. Gel prepolymer was prepared by combining 1/4 volume of 40% acrylamide, 1/67 volume of 2% BIS (Bio-Rad) and 1/100 volume of 2% red fluorescent carboxylate-modified beads (0.5 μm diameter, Invitrogen). A volume (1/200) of 10% ammonium persulfate and 1/2,000 volume of TEMED (Bio-Rad) were added to the prepolymer to initiate the polymerization. The mixture (25 μl) was pipetted immediately onto the activated glass substrate followed by placing a round coverslip (No. 1, 12 mm diameter; Fisher) onto the gel droplet. The dish was then turned upside down to allow the 0.5-μm fluorescent tracer particles to stay near the top of the gel during gelation. After 30 min, the coverslip was removed and the gel was washed with 50 mM HEPES buffer (pH 8.5). The gel surface was treated with 1 mM sulphosuccinimidyl-6-(4-azido-2-nitrophenylamino) hexanoate (Sulfo-SANPAH; Pierce) in HEPES buffer, exposed under ultraviolet light for 10 min, washed twice with HEPES solution, washed once with PBS and coated with collagen I (0.2 mg ml −1 , Invitrogen) in PBS at 4 °C overnight. Before cell seeding, the polyacrylamide gel dish was washed with PBS, sterilized by ultraviolet light for 10 min and immersed in DMEM solution without FBS for 1 h. For wounding the monolayer, a thin PDMS blocker was placed on the gel surface and MCF-7 cells were seeded on the exposed area. After 24 h of culture, the PDMS blocker was removed to create a cell-free region and initiate collective cell migration. Fluorescence imaging of registration particles and tracer particles near the leading edge was conducted before and after the application of 0.25% trypsin. The traction force distribution was estimated using a traction force microscopy algorithm in ImageJ [44] . Imaging and data analysis Cellular behaviour was monitored using a TE2000-U inverted fluorescence microscope from Nikon (Tokyo, Japan). Time-lapse phase contrast and fluorescence images were captured using a Photometric CCD camera (Tucson, AZ). All fluorescence images were taken with the same exposure time to compare the relative fluorescence intensity. Time-lapse videos were obtained via images taken at 5-min intervals. Imaging analysis was performed using ImageJ. Statistical analysis Data are presented as mean±s.e.m. Experiments were performed in triplicate and repeated at least three times independently. Student’s t -tests were performed to compare experimental groups. For comparing multiple groups, a one-way analysis of variance and Tukey’s post hoc test were used. Statistically significant P values were assigned as follows: * P <0.05, ** P <0.01 or *** P <0.001. To determine the spatial distribution of leader cells, histograms of cell intensity were determined for each row of cells parallel to the leading edge. Each row was 25 μm in width and over 200 cells were measured. How to cite this article: Riahi, R. et al. Notch1–Dll4 signalling and mechanical force regulate leader cell formation during collective cell migration. Nat. Commun. 6:6556 doi: 10.1038/ncomms7556 (2015).